Interplay between the Kondo effect and the Ruderman–Kittel–Kasuya–Yosida interaction The interplay between the Ruderman–Kittel–Kasuya–Yosida interaction and the Kondo effect is expected to provide the driving force for the emergence of many phenomena in strongly correlated electron materials. Two magnetic impurities in a metal are the smallest possible system containing all these ingredients and define a bottom-up approach towards a long-term understanding of concentrated/dense systems. Here we report on the experimental and theoretical investigation of iron dimers buried below a Cu(100) surface by means of low-temperature scanning tunnelling spectroscopy combined with density functional theory and numerical renormalization group calculations. The Kondo effect, in particular the width of the Abrikosov–Suhl resonance, is strongly altered or even suppressed due to magnetic coupling between the impurities. It oscillates as a function of dimer separation revealing that it is related to indirect exchange interactions mediated by the conduction electrons. Magnetic atoms embedded in a non-magnetic host metal have been intensively studied in solid state physics during the last decades. At low temperature, these systems can exhibit strong electronic correlations that give rise to various fascinating phenomena beyond the single particle picture [1] . The magnetic impurities, elements with partially filled d or f orbitals, have localized spins that interact with the surrounding conduction electrons. Below a characteristic temperature T k , the coupling between conduction electrons and the localized spins leads to the Kondo effect, a collective screening of the impurity spins. Since the impurities are coupled to the same conduction electrons, a magnetic interaction between impurities leading to magnetic ordering may arise. This indirect exchange interaction is well known as Rudermann–Kittel–Kasuya–Yosida (RKKY) interaction [2] , [3] , [4] . Many phenomena in strongly correlated electron physics, especially for heavy-fermion metals such as unconventional superconductivity or quantum critical behaviour are attributed to the competition of RKKY interaction with Kondo physics [5] . While single-impurity Kondo physics, where the impurities can be treated individually, has been studied for a long time in macroscopic measurements [6] and more recently in nanostructures [7] , [8] , [9] , [10] , [11] , [12] , [13] , [14] , [15] , [16] , [17] , [18] a detailed knowledge of the transition towards a systems of interacting impurities is still lacking. Although, the concept of spatially extended indirect exchange in the two-impurity Kondo problem is well established in theoretical research, experimental studies report a rather short-ranged interaction between Kondo impurities. Scanning tunnelling spectroscopy of two magnetic atoms adsorbed on a noble metal surface found a significant change of Kondo features only for small dimer distances, for example, a few angstroms [19] , [20] , [21] , [22] . Attaching two magnetic atoms at the ends of a non-magnetic chain may enhance the range of the magnetic exchange interaction [23] , but structural relaxation in these nanostructures make it difficult to compare different chain lengths with each other. Furthermore, this approach is limited towards certain directions and hence gives no access to all possible discrete separations on a surface. Two interacting Kondo impurities can also be realized by two coupled quantum dots [24] , [25] . However, owing to geometrical constraints, the spatial dependence of the interaction strength cannot be studied in these experiments. Recent studies showed that the short distance regime can be experimentally explored by atomic point contacts [26] . Here we address the transition from a single Kondo impurity towards a coupled system and investigate experimentally as well as theoretically the interaction between two magnetic impurities. In particular, the study of spatial extension and strength of the RKKY interaction in a bulk system, as reported here, may help to develop a broader understanding of strongly correlated electron systems. Iron dimers below a copper surface In our experiment, we investigate single isolated magnetic Fe dimers buried below the Cu(100) surface with a low-temperature scanning tunnelling microscope (see Methods section). We have chosen Fe in copper (Cu) because of its low Kondo temperature [16] . Furthermore, in this work, we focus on dimers located in the fifth Cu monolayer below the surface [17] owing to two reasons. First, we are interested in bulk impurities, and for dimers located within the first monolayers the presence of the surface may strongly influence the magnetic interaction. Second, for much deeper impurity positions, the energy dependence of the band structure itself may cause strong spectroscopic signatures around the Fermi energy that make it hard to extract microscopic information of the Kondo system [27] . In our experiment dimers can be identified by their topographic signature. When two Fe atoms are very close to each other their interference pattern starts to overlap. The dimer configuration within the atomic lattice can be extracted by analysing the topography ( Supplementary Note 1 and Supplementary Fig. 1 ). As a first striking example Fig. 1 depicts that two adjacent Fe impurities that are separated by R =0.57 nm show a considerably different spectral signature compared with a single impurity. For a tip position direct at the centre of the interference pattern of the dimer a narrow peak is found in the background subtracted differential conductance Δd I /d V (see Methods section). For equivalent spatial positions on the interference pattern of the dimer and of the monomer ( Fig. 1a,b , respectively) nearly the same line shape is observed ( Fig. 1c ). A closer look at the spectroscopic data, however, reveals two main differences. At first, the signature found in the centre of the standing-wave pattern of the dimer (purple dots) is twice as high as the signature with a tip position at the border (blue dots). This feature can be explained by the vicinity of the second Fe impurity that induces the same signature at the centre as the first one. More significantly, the resonance width for the dimer is broadened compared with a monomer (blue and green dots), while the line shape as well as the amplitude is nearly the same for both spectra. Up to now there exists no fit formula or model for a magnetic dimer in an STM experiment taking into account the electron propagation of the material and all different scenarios that may occur in the system. Our many-body calculations (see below), however, suggest that the same fit formula as for the single-impurity case also describes the spectral signature of two interacting impurities (see Supplementary Fig. 2 and Supplementary Note 2 ). We use a fit formula based on the model of Újsághy et al. [28] , but replace the Lorentzian form of the Kondo resonance by a phenomenological form of the Kondo resonance proposed by Frota et al. [29] , [30] The final expression correctly describes Kondo features such as line shape [31] and more markedly the phase shift caused by the resonance fairly well in both experiment and many-body calculations [16] , [17] , [32] , [33] . By fitting the spectroscopic signal of the dimer, the half-width at half-maximum Δ of the Kondo resonance of 16.5±1.5 and 15.0±3.6 mV is extracted with a tip position at the centre and at the border, respectively. Both values are nearly the same and slightly but significantly higher than the resonance width Δ=12.2±2.3 mV observed for the single Fe impurity. Please note that the data for the monomer and dimer was measured with the same tip on the same sample, so that the observed differences in the spectroscopic signature are not related to tip properties. 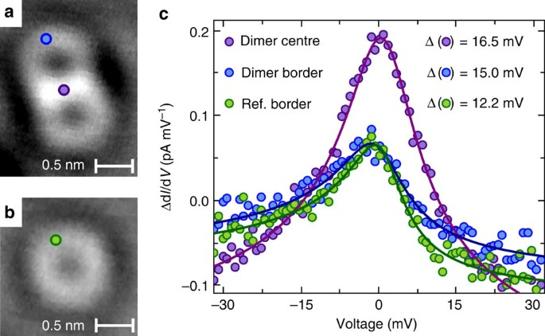Figure 1: Comparison of an iron dimer with an isolated single impurity located in the same monolayer. (a) STM constant current topographies of a dimer with a separation ofR=0.57 nm, and (b) a monomer. (c) Single ΔdI/dVspectra for different lateral tip positions, marked in the topographies by circles. The solid curves show fits to the spectra. At the centre of the interference pattern of the dimer (purple dots) a peak-like feature is observed. Compared with the monomer, the half-width at half-maximum (HWHM) of the Kondo resonance Δ is increased. More clearly this effect can be seen in spectra with the same lateral tip positions (green and blue dots). The resonance width of the dimer is broadened, while the line shape as well as the amplitude is nearly the same for both spectra. Image parameters are as follows: (a,b)V= −31 mV andI=0.2 nA, colour scale from −4.0 pm (black) to 5.5 pm (white). Spectroscopy parameters are as follows: (c)VSP= −40 mV andISP=0.3 nA. Figure 1: Comparison of an iron dimer with an isolated single impurity located in the same monolayer. ( a ) STM constant current topographies of a dimer with a separation of R =0.57 nm, and ( b ) a monomer. ( c ) Single Δd I /d V spectra for different lateral tip positions, marked in the topographies by circles. The solid curves show fits to the spectra. At the centre of the interference pattern of the dimer (purple dots) a peak-like feature is observed. Compared with the monomer, the half-width at half-maximum (HWHM) of the Kondo resonance Δ is increased. More clearly this effect can be seen in spectra with the same lateral tip positions (green and blue dots). The resonance width of the dimer is broadened, while the line shape as well as the amplitude is nearly the same for both spectra. Image parameters are as follows: ( a , b ) V = −31 mV and I =0.2 nA, colour scale from −4.0 pm (black) to 5.5 pm (white). Spectroscopy parameters are as follows: ( c ) V SP = −40 mV and I SP =0.3 nA. Full size image Different dimer configurations In order to obtain deeper insights into the interaction of two Kondo atoms with each other, an overview of different iron dimer configurations with their corresponding spectroscopic signature is presented in Fig. 2 . All dimers ( Fig. 2a–e ) are located in the fifth monolayer and the interatomic distance R between adjacent iron atoms ranges from R =0.51 to 1.02 nm ( Fig. 2f–j ). For the most compact dimer configuration, no signature of the Kondo effect is observed ( Fig. 2k and Supplementary Figs 3 and 4 ). Further details of this configuration are discussed in Supplementary Note 3 . With increasing interatomic distance features at the Fermi energy owing to the Kondo effect are found ( Fig. 2l–o ). All signatures can be fairly well described by the phenomenological fit formula. The different configurations show a variation of the Kondo resonance width Δ, depicted in Table 1 (a complete set of fit parameters is provided in Supplementary Table 1 ). 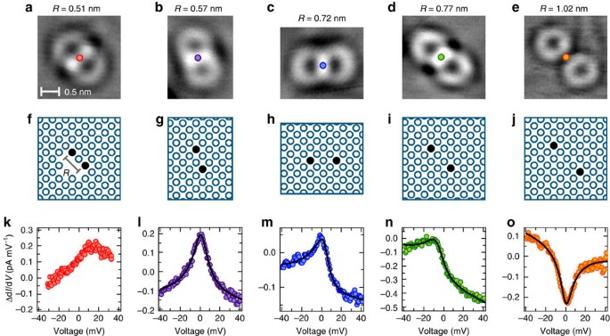Figure 2: Overview of different dimer configurations. All dimers are situated in the fifth monolayer below the Cu(100) surface. (a–e) Constant current topographies of different dimer configurations with increasing distance. (f–j) Corresponding atomic configurations. (k–o) Single ΔdI/dVspectra (dots) with a tip position at the centre of the standing-wave pattern. The solid curves show fits to the spectra. While for the smallest dimer configuration (f) no feature around zero bias is observed, all other configurations (g–j) show Kondo fingerprints. The solid black curves show fits to the spectra. Image parameters are as follows: (a–e)V=−31 mV andI=0.2 nA, colour scale from −4.0 pm (black) to 5.5 pm (white). Spectroscopy parameters are as follows: (k)VSP=−31 mV andISP=0.25 nA; (l,n)VSP=−40 mV andISP=0.3 nA; (m,o)VSP= −40 mV andISP=0.25 nA. Figure 2: Overview of different dimer configurations. All dimers are situated in the fifth monolayer below the Cu(100) surface. ( a – e ) Constant current topographies of different dimer configurations with increasing distance. ( f – j ) Corresponding atomic configurations. ( k – o ) Single Δd I /d V spectra (dots) with a tip position at the centre of the standing-wave pattern. The solid curves show fits to the spectra. While for the smallest dimer configuration ( f ) no feature around zero bias is observed, all other configurations ( g – j ) show Kondo fingerprints. The solid black curves show fits to the spectra. Image parameters are as follows: ( a – e ) V =−31 mV and I =0.2 nA, colour scale from −4.0 pm (black) to 5.5 pm (white). Spectroscopy parameters are as follows: ( k ) V SP =−31 mV and I SP =0.25 nA; ( l , n ) V SP =−40 mV and I SP =0.3 nA; ( m , o ) V SP = −40 mV and I SP =0.25 nA. Full size image Table 1 Kondo effect as function of dimer separation. Full size table All values are increased compared with a single iron impurity that exhibits a resonance width of Δ 0 =11.7±3.0 mV. This value is obtained by averaging over different measurements with different tips and lateral tip positions. Remarkably, the resonance width found for the different dimers is not a monotonic function of their interatomic distance. While for R =0.57 and 0.72 nm, the width of the Kondo resonance is slightly increased, a separation of R =0.77 nm shows a value that is nearly two times larger compared with the single-impurity value. For larger separation of R =1.02 nm, the resonance width decreases recovering nearly the single-impurity reference value. The experimental findings can be understood within the two-impurity Kondo model (TIKM), the simplest theoretical model to describe magnetic interactions between Kondo impurities [34] , [35] , [36] . The qualitative ground-state properties of the TIKM can be derived by considering the two competing effects ( Fig. 3a ). On the one hand is the single-impurity Kondo effect that tries to screen each impurity spin independently, and on the other hand is the magnetic interaction between the impurities, promoting a non-local correlation between the localized spins. 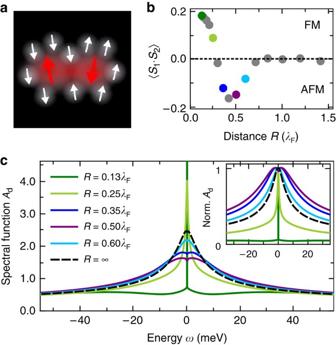Figure 3: Competition of Kondo effect and magnetic exchange interaction between two impurities. (a) Schematic view of the two-impurity Kondo model, illustrating the screening of the local moments (red arrows) by the itinerant conduction electrons (white arrows). Since both impurities are coupled to the same conduction electrons a magnetic exchange interactionJexarises intrinsically between the two-impurity spins (S1andS2). (b) The spin–spin correlation function of the localized moments shows an oscillation between FM and AFM coupling as function of their distanceR(given in multiples of the Fermi wavelengthλF). (c) Evolution of the spectral functionAdof the two-impurity Kondo model for different distances. The inset shows the normalized (norm) spectral function with respect to their value at the Fermi energy. Figure 3: Competition of Kondo effect and magnetic exchange interaction between two impurities. ( a ) Schematic view of the two-impurity Kondo model, illustrating the screening of the local moments (red arrows) by the itinerant conduction electrons (white arrows). Since both impurities are coupled to the same conduction electrons a magnetic exchange interaction J ex arises intrinsically between the two-impurity spins ( S 1 and S 2 ). ( b ) The spin–spin correlation function of the localized moments shows an oscillation between FM and AFM coupling as function of their distance R (given in multiples of the Fermi wavelength λ F ). ( c ) Evolution of the spectral function A d of the two-impurity Kondo model for different distances. The inset shows the normalized (norm) spectral function with respect to their value at the Fermi energy. Full size image Spectral properties of the TIKM can be obtained for T =0 K by using numerical renormalization group (NRG) calculations [37] . Here, we use as model for the Cu host a free electron gas with Fermi wavelength k F and other model parameters such that the individual impurities are well in the Kondo regime (see Methods section). No direct exchange is included, that is, only RKKY-generated spin correlations are considered. This is in good agreement with the experiment as the iron atoms are well separated such that direct coupling can be neglected. Varying the inter-impurity distance R , we first observe in Fig. 3b the expected oscillation of the spin–spin correlation function, reflecting the corresponding behaviour of the RKKY interaction [36] . Note that the correlations decay rapidly on a scale of the Fermi wavelength λ F , and start out antiferromagnetic (AFM) as the impurities approach each other, becoming ferromagnetic (FM) as the separation drops below one quarter of the Fermi wavelength. The corresponding spectral functions are collected in Fig. 3c . As expected, they resemble the spectra of independent impurities for large R , showing the particular hallmark of the many-body singlet state, a narrow resonance at the Fermi energy. With decreasing R , in the regime of AFM correlations, we observe an enhanced width, which is most apparent from the inset to Fig. 3c , where the spectra are normalized to their value at the Fermi energy. Similar results were obtained recently by applying perturbation theory [38] . In general, starting from well-separated impurities, one expect first an increase of the half-width at half-maximum Δ of the Kondo resonance for AFM correlations, showing a maximum for the configuration with the strongest AFM coupling. For small distances, FM coupling takes over leading to a reduction of Δ. This situation is similar to multi-orbital Kondo physics increasing the total spin of the system, which results in a strongly reduced Kondo scale [39] , [40] . As details of the Cu band structure cannot be included in the many-body calculation, we use first-principles calculations (see Methods section) to link the experimental findings to our model. The observed width of the Kondo resonance ( Fig. 4a ) and the calculated magnetic interaction strength J ex ( Fig. 4b ) have the same oscillation period. We are aware that ab initio calculations do not include correlations necessary to describe the Kondo effect and that many-body effects can alter the strength of the RKKY interaction. However, density functional theory (DFT) fairly well describes the electronic properties of the Cu substrate, that is, its Fermi surface, which is the main ingredient for such long-range magnetic exchange interactions and, in particular, the oscillation wavelength. 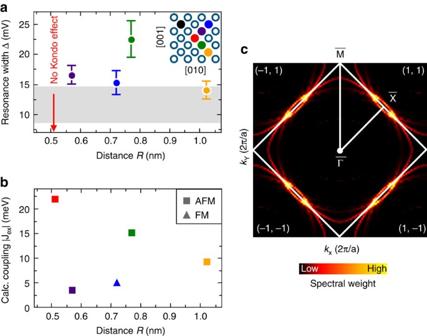Figure 4: Distance dependence and magnetic exchange coupling. (a) Observed Kondo resonance width Δ as function of the dimer separationR. The corresponding atomic configurations within the fifth monolayer are shown in the inset (black dot: position of the first Fe atom, colour dot: position of the second Fe atom). As reference, the averaged value for a single isolated fifth monolayer Fe impurity Δ0=11.7±3.0 mV is highlighted in light grey. Error bars resemble the 95 % confidence interval of the resonance width obtained by the fit. (b) Absolute calculated values for the exchange interaction |Jex| between two iron atoms below the Cu(100) surface. FM configurations are marked as triangles, whereas AFM configurations as squares. (c) Bloch spectral function at the Fermi energy projected on the layer in which the impurities are embedded. The two-dimensional Fermi energy contours are of almost square-like shape with flat regions along the directions, which is reminiscent of the bulk Fermi surface of Cu projected on the plane perpendicular to the (100) direction. Figure 4: Distance dependence and magnetic exchange coupling. ( a ) Observed Kondo resonance width Δ as function of the dimer separation R . The corresponding atomic configurations within the fifth monolayer are shown in the inset (black dot: position of the first Fe atom, colour dot: position of the second Fe atom). As reference, the averaged value for a single isolated fifth monolayer Fe impurity Δ 0 =11.7±3.0 mV is highlighted in light grey. Error bars resemble the 95 % confidence interval of the resonance width obtained by the fit. ( b ) Absolute calculated values for the exchange interaction |J ex | between two iron atoms below the Cu(100) surface. FM configurations are marked as triangles, whereas AFM configurations as squares. ( c ) Bloch spectral function at the Fermi energy projected on the layer in which the impurities are embedded. The two-dimensional Fermi energy contours are of almost square-like shape with flat regions along the directions, which is reminiscent of the bulk Fermi surface of Cu projected on the plane perpendicular to the (100) direction. Full size image For the smallest separation with R =0.51 nm (red configuration), an AFM exchange coupling with J ex =−21.8 meV is predicted. Here no Kondo signature around zero bias is found in the experiment. The AFM coupling between the localized impurity spins seems to be stronger than the coupling to the surrounding conduction electrons and hence the Kondo effect is suppressed. A slightly weaker AFM exchange interaction of J ex =−15.2 meV is calculated for a distance R =0.77 nm (green configuration), experimentally showing the strongest broadening. Configurations R =0.57 and 1.02 nm exhibit smaller magnetic exchange interaction J ex and hence cause a smaller broadening. Following the simulation, a FM coupling is expected for a separation of R =0.72 nm. According to the TIKM, this leads to a reduction of the Kondo resonance width, but experimentally an increased value is found. Although an enhancement of the Kondo resonance width for a FM-coupled dimer would be a quite interesting and unexpected new result, we think that based on our current results a substantial statement on that cannot be given. In most calculations and in ours as well, the ground state of the Kondo system ( T =0 K) is calculated but in general the (experimental) temperature plays a crucial role. We know that the Kondo temperature T k for single isolated Fe impurities is ~18 K (ref. 16 ). In the experiment, we are restricted to T =6 K, which means that we are in the low-temperature limit T < T k for a single Fe impurity and for AFM-coupled dimers as the Kondo resonance is expected to broaden for this type of coupling. Here, the experimental results can be directly compared with the calculations. As the resonance width reduces for FM coupling according to our model, this assumption is no longer true. It is well known [1] and also observed experimentally [13] , [41] that the resonance intrinsically broadens going to finite temperature ( T > T k ). Experimentally, the ground-state properties can then only be extracted by going to lower temperature. Spatial dependence of the RKKY interaction A detailed analysis of our results reveals a strong directional dependence of the exchange interaction ( Supplementary Fig. 5 ). Both theory and experiment highlight that the direction promotes the strongest magnetic coupling between impurities. Compare, for example, the red with the purple dimer configuration (or the green with the blue one). Here the distance between the iron atoms is nearly the same, but J ex is stronger for the dimer oriented along the direction. This feature was also observed for magnetic dimers on a metal surface [42] , [43] and may be explained by an aliasing between the periodicity of the lattice and the wavelength of the RKKY oscillation. As the RKKY interaction is mediated by the conduction electrons also anisotropies in the band structure can cause a directional dependence. Cu is well known to show strong directional Friedel oscillations with wave vectors and amplitudes depending on the crystal direction [17] , [44] , [45] , [46] , [47] . Indeed, the two-dimensional spectral function projected on the fifth layer below the surface ( Fig. 4c ) highlights the Fermi energy contours weighted with the electronic occupation. Interestingly a squared-like shape is obtained with flat regions perpendicular to the diagonals. This is the required ingredient to obtain a strong focusing effect of the electronic beams mediating the magnetic exchange interactions among the impurities. The shape obtained is reminiscent of the energy contour obtained in the bulk of Cu. Interestingly, our simulations demonstrate that once the impurities are put on top of the surface or embedded in the surface, the magnetic exchange interactions decrease strongly since the corresponding bulk energy contours lose their intensity ( Supplementary Note 4 and Supplementary Fig. 6 ). Many of the experimental and theoretical results presented here for dimers located in the fifth monolayer are also obtained for dimers located in other monolayers, indicating that the RKKY interaction is only slightly affected by the presence of the surface ( Supplementary Fig. 7 ). Our experimental findings are therefore not only relevant for artificially nanostructures but also may be relevant for the investigation of strongly correlated bulk systems including a crossover from local Kondo screening of the constituents to the formation of magnetic ordering. Being able to measure the properties of two magnetic bulk impurity is a prerequisite for the understanding and design of more complex structures. For example, trimers or linear chains are promising model systems for a bottom-up approach towards materials in which the local moments are arranged in a periodic array, so-called Kondo lattices. Up to now, theoretical models describing these systems are mainly isotropic and mostly consider only nearest or next nearest neighbour magnetic interactions. This work illustrates that the RKKY interaction between two bulk Kondo impurities can be significantly large also for greater distances and furthermore shows strongly directional behaviour. For iron dimers in Cu, the RKKY interaction can increase the Kondo resonance width by a factor of two for a separation that is more than twice the length of the unit cell. As bulk impurities are well known to show universal behaviour to a certain extent, we expect that magnetic interactions at larger distances may be significant also in other systems. Future experimental and theoretical work will focus on how multi-orbital Kondo physics and magnetic anisotropy affect the RKKY interaction. In general, for Fe in Cu deviations from a coupled spin 1/2 model might be expected but within our current spectral resolution (experimental temperature), we are not able to circumstantiate any differences. Whether the experimental observation of line broadening for the FM configuration is linked to this or mainly owing to thermal broadening has to be tested by future work. From an experimental point of view, systems with a lower Kondo temperature may give further insights as these systems are more strongly affected by spin–orbit coupling and crystal-field splitting [13] , [18] . Manganese or rare earth impurities are interesting candidates for such an experiment. Scanning tunnelling microscopy and spectroscopy The STM experiments presented here were performed using a home-built low-temperature scanning tunnelling microscope operating at 6 K at pressures below 5 × 10 −11 mbar. The Cu(100) single-crystal substrate is cleaned by several cycles of argon bombardment and electron beam heating. A Cu alloy with a small amount (~0.04%) of iron impurities is prepared through simultaneous deposition of Cu and iron from two electron beam evaporators. We use electrochemically etched tungsten tips, prepared by annealing and argon ion bombardment. The performance of the tip is tuned by controlled voltage pulses and smooth tip-sample contacts. The x - and y axis in the constant current topographies are aligned to the [010] and [001] crystallographic direction, respectively. Differential conductance measurements are obtained using a lock-in technique adding a modulation of 1.4–2.0 mV to the sample voltage at a frequency of 2,190 Hz. The spectra are acquired by setting the tip height to give a set point current I SP at a set point voltage V SP , holding the tip at this fixed position above the surface, and then sweeping the voltage while recording d I /d V . The spectra are not sensitive on the impedance of the tunnelling junction. Typical differential conductance d I /d V spectra measured with a tip position above the interference pattern of a Fe impurity reveal a strong signature around zero-bias voltage, which is attributed to the Kondo effect and cannot be seen in spectra of the bare Cu surface. In order to remove artefacts that originate from the tip, we normalize the d I /d V data around an impurity by subtracting from the measured signal the spectra of the bare surface d I 0 /d V far away from the impurity [48] . NRG calculations Magnetic impurities in metals are conventionally described using a variant of the Anderson impurity model [1] . Here, we study the concrete model where we used standard notation for the different terms. The two magnetic impurities are located at sites R i , i=1, 2. Note that no explicit exchange between the impurities is included. To proceed, one introduces linear combinations, , for the impurity degrees of freedom. By this transformation, one obtains a model in which the states with even respectively odd parity couple via a hybridization function, to the corresponding band-electron degrees of freedom [49] . Assuming a free electron gas in D =3 for the band electrons, one can approximate this by and use a linearized dispersion for the explicit evaluation. Note that the relevant parameter to control the impurity distance in the model then becomes k F R 12 . Still, the model is a quantum impurity model that needs to be solved with a suitable numerical technique. We here use the NRG [37] that allows us to solve the two-impurity model at T =0 K in the Kondo regime. To that extent, we choose a value U /( π Γ 0 )=3 and ε d =− U /2. The NRG parameters were: discretization parameter Λ=2.5, 3,000 states per iteration kept with 100 NRG iterations in total. We calculated the spectral functions directly without using the self-energy. Please note that the many-body calculations can be described by a phenomenological form of the Kondo resonance proposed by Frota et al. [29] , [30] ; Supplementary Fig. 2 . Ab initio calculations The Korringa–Kohn–Rostoker Green function method [50] , [51] within the local-density approximation of the DFT is used to simulate and investigate the different Fe dimers embedded underneath the surface of Cu. The magnetic exchange interactions among Fe impurities were extracted using the frozen-potential approximation considering infinitesimal rotations of the magnetic moments [52] . As in the experiment, the iron impurities are located in the fifth monolayer below the Cu(100) surface. The magnetic exchange interaction J ex between two magnetic moments has been extracted by mapping the ab initio calculations to the Heisenberg model The magnetic exchange interaction J ex describes the coupling between the localized impurity spins and with and being their unit vectors. How to cite this article : Prüser, H. et al. Interplay between Kondo effect and Ruderman–Kittel–Kasuya–Yosida interaction. Nat. Commun. 5:5417 doi: 10.1038/ncomms6417 (2014).